The cleavage pattern of TDP-43 determines its rate of clearance and cytotoxicity TAR DNA-binding protein of 43 kDa (TDP-43) and its C-terminal fragment of 25 kDa (CTF25) play critical roles in amyotrophic lateral sclerosis and frontotemporal lobar degeneration. Although the overexpression of TDP-43 in cultured cells and animals results in the production of CTF25, the cleavage site that generates CTF25 and biological significance of the cleavage remain undetermined. Here we identify Asp174 as a cleavage site for CTF25. TDP-43 is cleaved initially after Asp174, which activates caspase-3/7 to accelerate TDP-43 fragmentation. Consequently, blockage of this cleavage results in a severe delay in TDP-43 clearance and prolonged necrotic cell death. We further show that the endoplasmic reticulum membrane-bound caspase-4 is the enzyme responsible for the cleavage after Asp174 and inhibition of caspase-4 activity slows TDP-43 fragmentation and reduces cell viability. These findings suggest that caspase-4-mediated cleavage after Asp174 is an initiator of TDP-43 clearance, which is required to avoid cell death induced by overexpressed TDP-43. Amyotrophic lateral sclerosis (ALS) is one of the most devastating neurodegenerative diseases and is characterized by muscle weakness due to the degeneration of both upper and lower motor neurons. Although the pathogenic mechanism of ALS remains unresolved, the RNA-binding protein TDP-43 has been shown to accumulate in cytoplasmic inclusions in the affected regions of the spinal cord and brain in patients with ALS and frontotemporal lobar degeneration (FTLD), respectively [1] , [2] . Subsequently, mutations linked with ALS and FTLD have been identified in the gene that encodes TDP-43, which has confirmed the significance of TDP-43 in the pathogenesis of these diseases [3] , [4] . Most of these mutations occur within or near the carboxyl-terminal (C-terminal) glycine-rich domain (GRD) of TDP-43, except for the D169G point mutation that resides in RNA recognition motif 1 (refs 3 , 4 ). TDP-43 is normally localized predominantly in the nucleus. However, in ALS and FTLD patients with TDP-43-positive cytoplasmic inclusions, the protein is abnormally phosphorylated, ubiquitinated and truncated. This results in the accumulation of an ~25-kDa C-terminal fragment (CTF25), in addition to other minor CTFs and the full-length TDP-43, in cytoplasmic aggregates. CTFs are hallmarks of forms of disease whose pathology is associated exclusively with abnormalities in TDP-43 and are observed in patients with not only ALS and FTLD but also Alzheimer’s disease [5] . Amino-terminal (N-terminal) analysis of CTFs obtained from brain autopsies of patients with FTLD has resulted in the identification of three cleavage sites, Arg208, Asp219 and Asp247, which give rise to CTFs [6] , [7] . However, the expected sizes of the resulting CTFs are less than 25 kDa, which suggests that CTF25 is probably cleaved at a different position. TDP-43 is a widely expressed 414-amino acid (a.a.) protein comprised of two RNA recognition motifs (RRM1 at a.a. 106–176 and RRM2 at a.a. 191–262) and the GRD [8] , [9] . The chronic stabilization of wild-type TDP-43 provokes cytotoxicity in cultured cells [10] . Transgenic mice expressing wild-type human TDP-43 also develop an ALS-like phenotype in a TDP-43 dose-dependent manner [11] . Finally, the expression of full-length wild-type human TDP-43 in the eyes of Drosophila leads to neurodegeneration, but a mutant that comprises only the C-terminal region from a.a. 202 does not have this effect [12] . The evidence listed above indicates that the increased expression of full-length TDP-43 is deleterious for neuronal survival. Therefore, the elucidation of mechanisms that underlie the clearance of TDP-43 is pivotal for understanding the pathogenesis of ALS and FTLD. Overexpression of TDP-43 in cultured cells and animals causes fragmentation of the protein, generating a 35-kDa C-terminal fragment (CTF35) and CTF25 (refs 11 , 13 , 14 , 15 ). Although the associated N-terminal fragments (NTFs) of TDP-43 are degraded quickly, the CTFs form aggregates that can also contain full-length TDP-43. CTF35 is generated by caspase-3/7-mediated cleavage after Asp89, which is embedded in the consensus caspase-recognition motif [13] , [14] , [15] , [16] . Initially, Asp219 was suggested as the candidate cleavage site for CTF25; however, the estimated molecular weight of the fragment that comprises a.a. 220–414 is less than 25 kDa (refs 13 , 16 , 17 ). Subsequently, Asp169 was suggested as the cleavage site, but introduction of the mutation D169E does not inhibit the generation of CTF25 completely, which suggests the existence of a second CTF25 fragment [15] . Moreover, the knockout of caspase-3 does not prevent the generation of CTF25, which implies that at least a proportion of CTF25 is produced by a different mechanism from that by which CTF35 is generated [14] . However, the exact cleavage site of CTF25, the enzyme responsible and the biological significance of the cleavage remain undetermined. In this study, we found that CTF25 is comprised of two fragments of TDP-43, which are cleaved after Asp174 and Asp169, respectively, by different mechanisms. Pulse-chase analysis demonstrated that TDP-43 is cleaved initially after Asp174 to generate CTF25, before the production of CTF35 in a caspase-3/7-independent manner. This cleavage is required for the subsequent activation of caspase-3/7. The introduction of a cleavage-resistant mutation at Asp174 resulted in a severe delay in the clearance of full-length TDP-43 and prolonged necrotic cell death. Finally, we identified that endoplasmic reticulum (ER) membrane-bound caspase-4 was the enzyme responsible for the initial cleavage after Asp174. In accordance, CTF aggregates were formed initially at the ER and then ER stress was induced subsequently. Taken together, these findings suggest that caspase-4 monitors the amount of TDP-43 in the ER by recognizing Asp174 and when the ER is overloaded with TDP-43, caspase-4 cleaves a small portion of TDP-43. This cleavage triggers the downstream caspase-3/7 pathway, which reduces the full-length TDP-43-mediated cytotoxicity, a process that leads to necrosis, by promoting fragmentation. CTF25 is generated before CTF35 To clarify how TDP-43 is metabolized under physiological conditions in vivo , we first examined the fragmentation pattern of TDP-43 in multiple human cell lines under stress-free conditions. Although present in much smaller amounts than full-length TDP-43, two CTFs, namely CTF35 and CTF25, were observed in all of the cells examined ( Supplementary Fig. 1a ). This suggests that TDP-43 is degraded through a common mechanism that involves the generation of CTF35 and CTF25. Consequently, next we established a human U2OS-derived stable cell line that expressed wild-type TDP-43 tagged with SNAP-tag at the N terminus and a HaloTag at the C terminus (SNAP-TDP-43(WT)-HTC) under the control of Doxycycline (Dox) using the ‘Tet-On’ system. After the expression of SNAP-TDP-43(WT)-HTC had been induced for 24 h, we monitored the fragmentation of TDP-43 over time. The level of SNAP-TDP-43(WT)-HTC remained constant until 48 h, after which it decreased markedly. The induced protein was cleared almost completely at 120 h ( Fig. 1a ). During the time course of TDP-43 clearance, we observed three NTFs designated SNAP-N25, -N18 and -N8 and two CTFs designated C35-Halo and C25-Halo ( Fig. 1a ). 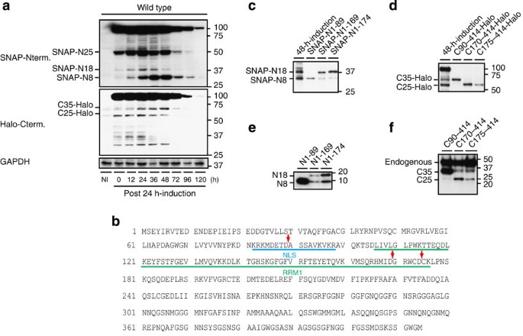Figure 1: Identification of the cleavage sites in TDP-43. (a) Transient expression of SNAP-TDP-43(WT)-HTC was induced with Dox for 24 h, and its metabolism was monitored at the indicated time points. The N terminus of TDP-43 was detected with an anti-SNAP-tag pAb and the C terminus of TDP-43 was detected with an anti-HaloTag pAb. GAPDH was used as the loading control. NI, no induction. (b) The entire amino-acid sequence of TDP-43 is shown, and the identified cleavage sites are indicated with red arrows. NLS, nuclear localization signal; RRM1, RNA recognition motif 1. SNAP-tagged NTFs (c) and Halo-tagged CTFs (d) were expressed transiently in U2OS cells. The resultant whole-cell lysates were subjected to western blot analysis with anti-SNAP-tag pAb (c) and anti-HaloTag pAb (d), respectively. Whole-cell lysate from U2OS cells in which the expression of SNAP-TDP-43(WT)-HTC had been induced for 48 h was loaded as a size control. Untagged NTFs (e) and CTFs (f) were expressed transiently in U2OS cells. The resultant whole-cell lysates were subjected to western blot analysis with anti-TDP-43 N terminus pAb (e) and anti-TARDBP pAb to detect the C-terminal region (f). Cterm, C-terminal; Nterm, N-terminal. Figure 1: Identification of the cleavage sites in TDP-43. ( a ) Transient expression of SNAP-TDP-43(WT)-HTC was induced with Dox for 24 h, and its metabolism was monitored at the indicated time points. The N terminus of TDP-43 was detected with an anti-SNAP-tag pAb and the C terminus of TDP-43 was detected with an anti-HaloTag pAb. GAPDH was used as the loading control. NI, no induction. ( b ) The entire amino-acid sequence of TDP-43 is shown, and the identified cleavage sites are indicated with red arrows. NLS, nuclear localization signal; RRM1, RNA recognition motif 1. SNAP-tagged NTFs ( c ) and Halo-tagged CTFs ( d ) were expressed transiently in U2OS cells. The resultant whole-cell lysates were subjected to western blot analysis with anti-SNAP-tag pAb ( c ) and anti-HaloTag pAb ( d ), respectively. Whole-cell lysate from U2OS cells in which the expression of SNAP-TDP-43(WT)-HTC had been induced for 48 h was loaded as a size control. Untagged NTFs ( e ) and CTFs ( f ) were expressed transiently in U2OS cells. The resultant whole-cell lysates were subjected to western blot analysis with anti-TDP-43 N terminus pAb ( e ) and anti-TARDBP pAb to detect the C-terminal region ( f ). Cterm, C-terminal; Nterm, N-terminal. Full size image To identify the N-terminal cleavage sites for C35-Halo and C25-Halo, we isolated the CTFs ( Supplementary Fig. 1b ), which were subjected to the Edman sequencing analysis. The N-terminal sequence of C35-Halo was ASSAV, which indicates that C35-Halo was generated by cleavage after Asp89, corresponding to the previously described cleavage site for CTF35 ( Fig. 1b ) [13] . In contrast, although the predominant N-terminal amino-acid sequence of C25-Halo was XKLPNS, a small amount of protein that began with the sequence GRWXD was also detected. Given that it is difficult to detect cysteine by the Edman method, we concluded that C25-Halo is comprised of two fragments that are generated by cleavage after Asp174 and Asp169, respectively ( Fig. 1b ). Next we expressed N- and C-terminal products that would be generated by cleavage at the three identified sites to compare the molecular sizes of these products with those of the naturally occurring TDP-43 fragments. SNAP-N1-89 was identical in molecular size to SNAP-N8, and C90-414-Halo was identical to C35-Halo ( Fig. 1c,d ). Furthermore, the molecular weights of the tag-free TDP-43(N1-89) and TDP-43(C90-414) proteins were nearly 8 and 35 kDa, respectively ( Fig. 1e,f ), which suggests that SNAP-N8 is probably the partner fragment of C35-Halo. Similarly, SNAP-N1-169 and SNAP-N1-174 were identical in molecular size to SNAP-N18, and C170-414-Halo and C175-414 were identical to C25-Halo ( Fig. 1c,d ). The tag-free TDP-43(N1-169) and TDP-43(N1-174) proteins were both nearly 18 kDa, whereas the tag-free TDP-43(C170-414) and TDP-43(C175-414) proteins were both almost 25 kDa ( Fig. 1e,f ). Taken together, we concluded that SNAP-N18 is probably the partner fragment of C25-Halo and that C25-Halo is CTF25 tagged with Halo. To distinguish the two forms of CTF25, we designated CTF25 cleaved after Asp169 as CTF25(D169) and that cleaved after Asp174 as CTF25(D174). Given that the HaloTag is ~33 kDa, we could not observe the partner fragments of SNAP-N25. Consequently, we currently do not know whether SNAP-25 was generated by a minor splicing event or its partner CTF was degraded quickly. Of note, C25-Halo was generated before C35-Halo just after induction ( Fig. 1a ). We can rule out the possibility that all C25-Halo was generated by a second cleavage of CTF35, because SNAP-N18 was also generated earlier than SNAP-N8 ( Fig. 1a ). This result suggests that CTF25 is produced independently of the generation of CTF35, at least in part. TDP-43 clearance requires initial cleavage after Asp174 Next we investigated the physiological significance of TDP-43 cleavage at the three sites. To avoid activation of the caspase pathway by transient chemical transfection of the expression constructs, we established three stable cell lines that expressed SNAP-TDP-43-HTC with a single point mutation (D89E, D169G or D174A) under the control of Dox. We found that introduction of the D89E mutation completely blocked the generation of CTF35 without any alteration in the timing of the first appearance of CTF25 ( Fig. 2a ). However, full-length SNAP-TDP-43-HTC with the D89E mutation was cleared significantly faster than the wild-type protein ( Fig. 2a,c ). These results suggest that the generation of CTF35 is dispensable for TDP-43 clearance. 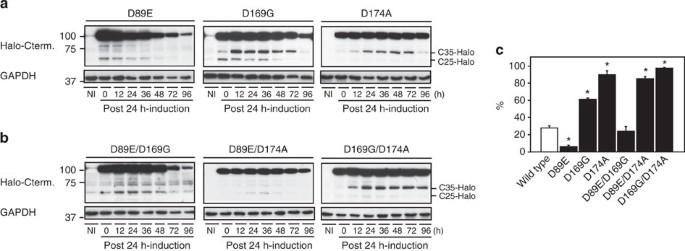Figure 2: Cleavage-resistant mutations affect the rate of clearance of full-length TDP-43. Transient expression of SNAP-TDP-43-HTC with the single point mutations D89E (left panel), D169G (middle panel) and D174A (right panel) (a) and that with the double mutations D89E/D169G (left panel), D89E/D174A (middle panel) and D169G/D174A (right panel) (b) was induced with Dox for 24 h. Subsequently, production of the CTFs indicated was monitored at the indicated time points. GAPDH was used as a loading control. NI, no induction. (c) The expression level of each full-length SNAP-TDP-43-HTC at 96 h relative to that at 0 h after induction for 24 h is plotted (Mann–WhitneyU-test, *P<0.05;n=6 for the wild type and 3 for all the mutants). Error bars represent the s.e.m. Cterm, C-terminal; GAPDH, glyceraldehyde 3-phosphate dehydrogenase. Figure 2: Cleavage-resistant mutations affect the rate of clearance of full-length TDP-43. Transient expression of SNAP-TDP-43-HTC with the single point mutations D89E (left panel), D169G (middle panel) and D174A (right panel) ( a ) and that with the double mutations D89E/D169G (left panel), D89E/D174A (middle panel) and D169G/D174A (right panel) ( b ) was induced with Dox for 24 h. Subsequently, production of the CTFs indicated was monitored at the indicated time points. GAPDH was used as a loading control. NI, no induction. ( c ) The expression level of each full-length SNAP-TDP-43-HTC at 96 h relative to that at 0 h after induction for 24 h is plotted (Mann–Whitney U -test, * P <0.05; n =6 for the wild type and 3 for all the mutants). Error bars represent the s.e.m. Cterm, C-terminal; GAPDH, glyceraldehyde 3-phosphate dehydrogenase. Full size image Similar to the D89E mutation, introduction of the D169G mutation had no effect on the timing of the appearance of CTF25 ( Fig. 2a ). However, the level of CTF25 was decreased slightly at 24 h as compared with the wild type. This was accompanied by a moderate reduction in the rate of clearance of full-length SNAP-TDP-43-HTC ( Fig. 2a,c ), which suggest that cleavage after Asp169 contributes to the efficient clearance of TDP-43 although it had little effect on the production of CTF25 during the early stages. In contrast, the production of CTF25 was inhibited almost completely by introduction of the D174A mutation, and more than 90% of the full-length SNAP-TDP-43-HTC remained at 96 h ( Fig. 2a,c ). These results suggest that TDP-43 is cleaved initially after Asp174 and blockage of this cleavage leads to the delayed clearance of full-length TDP-43. We further examined the significance of TDP-43 cleavage after Asp174 with respect to the initiation of TDP-43 clearance by introducing double mutations. The effect of the D89E/D169G mutation seemed to be the combined effect of the D89E mutation, which accelerates TDP-43 clearance, and the D169G mutation, which slows it down. Although the production of CTF35 was blocked, the timing of the first appearance of CTF25 by cleavage after Asp174 was not affected and full-length SNAP-TDP-43-HTC was cleared normally ( Fig. 2b,c ). In contrast, the introduction of D89E/D174A blocked the early production of CTF25 and only a small amount of CTF25 could be observed from 24 to 48 h ( Fig. 2b ). Similarly, the introduction of D169G/D174A completely inhibited the production of CTF25, which resulted in prolonged production of CTF35 ( Fig. 2b ). In both cases, more than 85% of the full-length SNAP-TDP-43-HTC remained at 96 h ( Fig. 2b,c ). Taken together, the results show that TDP-43 is cleaved initially after Asp174 to generate CTF25(D174) by a mechanism that is independent of the production of CTF35, and this cleavage is required for the onset of clearance of full-length TDP-43. In contrast, the cleavage after Asp169 contributes to TDP-43 clearance during later stages, although the amount of CTF25(D169) seems to be very low, at least in the soluble fraction. TDP-43 is phosphorylated during the later stages of turnover CTFs of TDP-43 are well known to be phosphorylated abnormally and form aggregates. To investigate the time course of insolubilization and phosphorylation of TDP-43, we separated the cell lysates obtained after the transient induction of SNAP-TDP-43(WT)-HTC into four fractions (TS buffer (TS)-soluble, Triton-X-100 (TX)-soluble, Sarkosyl (Sark)-soluble and Sark-insoluble) as described previously [7] . In contrast to the NTFs, which remained mainly in the soluble fractions, Sark-insoluble CTF35 and CTF25 were observed from 36 h and levels peaked at 72 h ( Fig. 3a and Supplementary Fig. 2 ). Subsequently, from 72 h, CTF35 and CTF25 were phosphorylated, which resulted in a slight shift to a higher molecular weight ( Fig. 3a ). In accordance with a previous study [18] , these results suggest the following pathway of TDP-43 turnover: initially, TDP-43 is cleaved, which generates CTFs, and then a proportion of the CTFs become insoluble and finally phosphorylated. 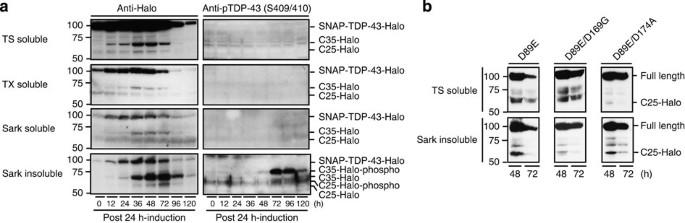Figure 3: Insolubilization and phosphorylation of CTFs are late events during the degradation of TDP-43. (a) Transient expression of SNAP-TDP-43(WT)-HTC was induced for 24 h in U2OS cells. The cell lysates collected at the indicated time points were separated into TS buffer (TS)-soluble, Triton-X-100 (TX)-soluble, Sarkosyl (Sark)-soluble and Sark-insoluble fractions. SNAP-TDP-43(WT)-HTC and its CTFs were detected with anti-HaloTag pAb (left panel) or with anti-phospho-TDP-43 (S409/410) pAb (right panel). (b) Transient expression of SNAP-TDP-43-HTC with the point mutation D89E (left panel), D89E/D169G (middle panel) and D89E/D174A (right panel) was induced for 24 h in U2OS cells. The cell lysates collected at the indicated time points were fractionated, and then SNAP-TDP-43-HTC and its CTFs in the TS-soluble and Sark-insoluble fractions were detected with anti-HaloTag pAb. Figure 3: Insolubilization and phosphorylation of CTFs are late events during the degradation of TDP-43. ( a ) Transient expression of SNAP-TDP-43(WT)-HTC was induced for 24 h in U2OS cells. The cell lysates collected at the indicated time points were separated into TS buffer (TS)-soluble, Triton-X-100 (TX)-soluble, Sarkosyl (Sark)-soluble and Sark-insoluble fractions. SNAP-TDP-43(WT)-HTC and its CTFs were detected with anti-HaloTag pAb (left panel) or with anti-phospho-TDP-43 (S409/410) pAb (right panel). ( b ) Transient expression of SNAP-TDP-43-HTC with the point mutation D89E (left panel), D89E/D169G (middle panel) and D89E/D174A (right panel) was induced for 24 h in U2OS cells. The cell lysates collected at the indicated time points were fractionated, and then SNAP-TDP-43-HTC and its CTFs in the TS-soluble and Sark-insoluble fractions were detected with anti-HaloTag pAb. Full size image Recent reports suggest that the oxidation of Cys173 and Cys175 promotes the aggregation of CTFs [19] , [20] , [21] . Given that Cys173 is more prone to oxidation than Cys175 (ref. 20 ), we examined the difference in insolubility between CTF25(D174) and CTF25(D169). The individual proteins were generated by the introduction of the D89E/D169G and D89E/D174A double mutations, respectively. CTF25(D174) was present at a substantial level in the soluble fractions but less was detected in the Sark-insoluble fractions ( Fig. 3b ). In contrast, CTF25(D169) was detected faintly in the soluble fractions, but more clearly in the Sark-insoluble fractions. These results suggest that CTF25(D169) is more prone to form insoluble aggregates than CTF25(D174). TDP-43-mediated cell death occurs before CTF aggregation Next we investigated how TDP-43 clearance affects cell viability. The expression of SNAP-TDP-43(WT)-HTC reduced cell viability slightly but significantly at 24 h post induction ( Fig. 4a,b ). Subsequently, cell viability reached a minimum value (~70%) at 48 h and recovered at 96 h. These results suggest that the onset of cell death induced by the overexpression of TDP-43 occurs earlier than the formation of CTF aggregates ( Figs 3a and 4a ). Introduction of the D89E mutation reduced the extent of cell death slightly ( Fig. 4a ), which correlated with the accelerated clearance of SNAP-TDP-43-HTC with the D89E mutation. In contrast, introduction of the D174A mutation, irrespective of the additional introduction of either the D89E or D169G mutation, resulted in more severe and prolonged cell death as compared with the wild-type protein ( Fig. 4a,b ). We also examined whether the cleavage-resistant mutations affected the viability of motor neurons derived from human embryonic stem cells (hESCs). The overexpression of SNAP-TDP-43(WT)-HTC reduced neuronal viability significantly ( Fig. 4c,d ). However, cell death was more severe in motor neurons that overexpressed SNAP-TDP-43-HTC with the D174A mutation ( Fig. 4d ). These results indicated that primary cleavage of TDP-43 after Asp174 was required to circumvent severe cell death. Interestingly, introduction of the D169G mutation also resulted in severe death, which was largely alleviated by additional introduction of the D89E mutation ( Fig. 4a,b,d ). This correlated with the moderately delayed clearance of full-length TDP-43, which was also alleviated by additional introduction of the D89E mutation ( Fig. 2a–c ). Therefore, although D169G mutation might affect cell survival by a mechanism that is distinct from the blockade of cleavage, the rate of clearance of full-length TDP-43 is at least one factor that influences cell survival, regardless of the amount of CTFs generated and the amount of aggregates that accumulate. 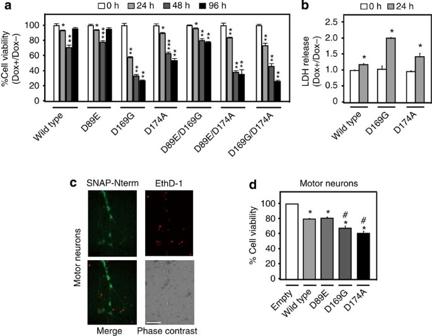Figure 4: Cleavage-resistant mutations affect cell death induced by the overexpression of TDP-43. Following induction of the expression of SNAP-TDP-43(WT)-HTC or the mutants indicated at the bottom in U2OS cells with Dox for 24 h, cell viability (a) and LDH release (b) were quantitated at the indicated time points. The cell viability (a) and the amount of LDH released (b) in the presence of Dox are plotted relative to those obtained in the absence of Dox (*P<0.05, **P<0.01, ***P<0.001;n=11 foraand 5 forb). Error bars represent the s.e.m. (c) Images of hESC-derived motor neurons that expressed SNAP-TDP-43(WT)-HTC whose N terminus was labelled with the SNAP ligand. Damaged cells were stained with EthD-1. The merged fluorescent image is presented in addition to the phase contrast image. Scale bars, 50 μm. (d) The viability of motor neurons that expressed SNAP-TDP-43(WT)-HTC or its mutants relative to that of motor neurons that were transducted with empty lentivirus (Empty) is plotted (mean±s.e.m.; *P<0.05, three independent experiments). Significant reductions in the viability of the cells that expressed the mutants compared with the cells that expressed SNAP-TDP-43(WT)-HTC are indicated by a hash (#P<0.05). The Mann–WhitneyU-test was used for all statistical analyses. Figure 4: Cleavage-resistant mutations affect cell death induced by the overexpression of TDP-43. Following induction of the expression of SNAP-TDP-43(WT)-HTC or the mutants indicated at the bottom in U2OS cells with Dox for 24 h, cell viability ( a ) and LDH release ( b ) were quantitated at the indicated time points. The cell viability ( a ) and the amount of LDH released ( b ) in the presence of Dox are plotted relative to those obtained in the absence of Dox (* P <0.05, ** P <0.01, *** P <0.001; n =11 for a and 5 for b ). Error bars represent the s.e.m. ( c ) Images of hESC-derived motor neurons that expressed SNAP-TDP-43(WT)-HTC whose N terminus was labelled with the SNAP ligand. Damaged cells were stained with EthD-1. The merged fluorescent image is presented in addition to the phase contrast image. Scale bars, 50 μm. ( d ) The viability of motor neurons that expressed SNAP-TDP-43(WT)-HTC or its mutants relative to that of motor neurons that were transducted with empty lentivirus (Empty) is plotted (mean±s.e.m. ; * P <0.05, three independent experiments). Significant reductions in the viability of the cells that expressed the mutants compared with the cells that expressed SNAP-TDP-43(WT)-HTC are indicated by a hash ( # P <0.05). The Mann–Whitney U -test was used for all statistical analyses. Full size image Caspase-4 is responsible for the cleavage after Asp174 Considering that all three cleavage sites are located after aspartic acid residues, we speculated that members of the caspase family were responsible for this cleavage. However, the amino-acid sequence around Asp174 does not contain a typical consensus caspase-recognition motif. Consequently, we performed an unbiased in vitro cleavage assay with recombinant human caspases (caspase-1 to -10). We found that caspases-3, -4, -6, -7, -8, -9 and -10 efficiently cleaved TDP-43, and all predominantly generated CTF35 ( Fig. 5a ). Introduction of the D89E mutation inhibited the production of this fragment completely, which indicated that seven caspases could cleave TDP-43 after Asp89 to generate CTF35 in vitro ( Fig. 5a ). On exposing the gel for a longer time, we observed CTF25 in samples treated with caspases-3, -4, -6, -7, -8 and -10, and probably caspase-9 ( Fig. 5a ). To characterize the cleavage site(s) of this fragment further, we introduced multiple point mutations. Introduction of the D89E mutation had no effect on the generation of CTF25, whereas the D89E/D169G/D174A triple mutation blocked it completely ( Fig. 5b ). Introduction of the D89E/D169G double mutation, on the other hand, reduced the amount of CTF25 generated by caspases-6 and -7 substantially and partially inhibited the caspase-3 and -8-dependent cleavage in vitro . In contrast, introduction of the D89E/D174A double mutation efficiently inhibited the production of CTF25 by caspases-4 and -10 and partially inhibited caspase-3 and -8-dependent cleavage ( Fig. 5b ). These results indicate that caspases-6 and -7 cleave predominantly after Asp169, whereas caspases-4 and -10 cleave predominantly after Asp174, resulting in the production of CTF25(D169) and CTF25(D174), respectively. In contrast, caspases-3 and -8 showed less specificity, recognizing both Asp169 and Asp174 in vitro , and caspase-9 did not generate CTF25 ( Fig. 5b ). 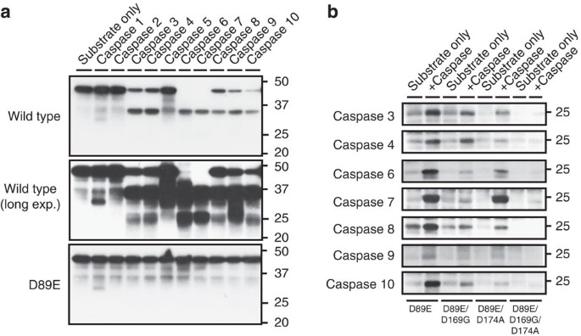Figure 5:In vitroassessment of caspases involved in TDP-43 fragmentation. (a) Wild-type TDP-43 (upper and middle panels) and the D89E mutant (lower panel) were synthesizedin vitroand incubated with each recombinant human caspase indicated at the top. The resultant mixture was subjected to western blot analysis with anti-TARDBP pAb. Long exp., long exposure. (b) The TDP-43 mutants indicated at the bottom were synthesizedin vitroand incubated with each recombinant human caspase indicated on the left. The resultant mixture was subjected to western blot analysis with anti-TARDBP pAb. Figure 5: In vitro assessment of caspases involved in TDP-43 fragmentation. ( a ) Wild-type TDP-43 (upper and middle panels) and the D89E mutant (lower panel) were synthesized in vitro and incubated with each recombinant human caspase indicated at the top. The resultant mixture was subjected to western blot analysis with anti-TARDBP pAb. Long exp., long exposure. ( b ) The TDP-43 mutants indicated at the bottom were synthesized in vitro and incubated with each recombinant human caspase indicated on the left. The resultant mixture was subjected to western blot analysis with anti-TARDBP pAb. Full size image To determine which caspases were responsible for the production of CTF35 and CTF25 in vivo , we examined the activation of all the candidate caspases indicated by the in vitro cleavage assay. We observed no activation of caspase-6, -8, -9 or -10 after the induction of SNAP-TDP-43(WT)-HTC. In contrast, caspases-3, -4 and -7 were activated efficiently but the enzymes followed different time courses ( Fig. 6a ). Caspase-3/7 were activated from 24 h and reached peak activity at 48 h. This time course is identical to that of the production of CTF35. In contrast, activation of caspase-4 was observed from the very early stages of TDP-43 induction and decreased gradually thereafter. The time at which caspase-4 is activated is identical to that at which CTF25 appears ( Fig. 6a ). Taken together, these results suggest that caspase-4 probably participates in the generation of CTF25(D174), whereas CTF35 is cleaved predominantly by caspase-3/7. 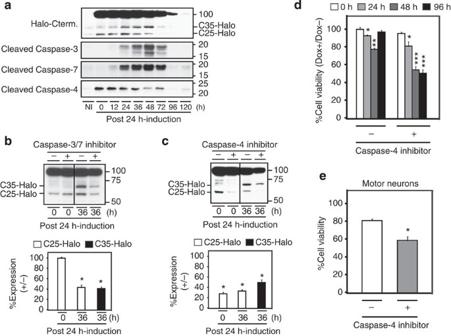Figure 6: Caspase-4 is responsible for the initial cleavage of TDP-43. (a) Transient expression of SNAP-TDP-43(WT)-HTC was induced with Dox for 24 h, and the activity of each caspase indicated on the left was monitored at the indicated time points. For comparative analysis, part of the same gel image obtained with anti-HaloTag pAb that was used inFig. 1ais shown at the top. NI, no induction. Transient expression of SNAP-TDP-43(WT)-HTC was induced with Dox for 24 h in the presence or absence of the caspase-3/7 inhibitor (b) or caspase-4 inhibitor (c). Then, the production of CTFs was monitored at the indicated time points. In the lower panels, the expression levels of the C35-Halo and C25-Halo fragments in the presence of the inhibitor relative to those in the absence of the inhibitor are plotted after normalization to the amount of full-length SNAP-TDP-43(WT)-HTC (*P<0.05;n=3). (d) Following induction of SNAP-TDP-43(WT)-HTC in U2OS cells for 24 h with Dox in the presence or absence of the caspase-4 inhibitor, cell viability was quantitated at the indicated time points. The cell viability with Dox relative to that without Dox is plotted (mean±s.e.m.; *P<0.05, **P<0.01, ***P<0.001;n=6 for 0 h and 12 for 24, 48 and 96 h). (e) The viability of hESC-derived motor neurons that expressed SNAP-TDP-43(WT)-HTC in the presence or absence of the caspase-4 inhibitor is plotted (mean±s.e.m.; *P<0.05, three independent experiments). The Mann–WhitneyU-test was used for all statistical analyses. Cterm, C-terminal. Figure 6: Caspase-4 is responsible for the initial cleavage of TDP-43. ( a ) Transient expression of SNAP-TDP-43(WT)-HTC was induced with Dox for 24 h, and the activity of each caspase indicated on the left was monitored at the indicated time points. For comparative analysis, part of the same gel image obtained with anti-HaloTag pAb that was used in Fig. 1a is shown at the top. NI, no induction. Transient expression of SNAP-TDP-43(WT)-HTC was induced with Dox for 24 h in the presence or absence of the caspase-3/7 inhibitor ( b ) or caspase-4 inhibitor ( c ). Then, the production of CTFs was monitored at the indicated time points. In the lower panels, the expression levels of the C35-Halo and C25-Halo fragments in the presence of the inhibitor relative to those in the absence of the inhibitor are plotted after normalization to the amount of full-length SNAP-TDP-43(WT)-HTC (* P <0.05; n =3). ( d ) Following induction of SNAP-TDP-43(WT)-HTC in U2OS cells for 24 h with Dox in the presence or absence of the caspase-4 inhibitor, cell viability was quantitated at the indicated time points. The cell viability with Dox relative to that without Dox is plotted (mean±s.e.m. ; * P <0.05, ** P <0.01, *** P <0.001; n =6 for 0 h and 12 for 24, 48 and 96 h). ( e ) The viability of hESC-derived motor neurons that expressed SNAP-TDP-43(WT)-HTC in the presence or absence of the caspase-4 inhibitor is plotted (mean±s.e.m. ; * P <0.05, three independent experiments). The Mann–Whitney U -test was used for all statistical analyses. Cterm, C-terminal. Full size image Next we examined how the activation of each caspase was affected by the introduction of cleavage-resistant mutations. Introduction of the D89E mutation did not affect the timing of caspase-4 activation ( Supplementary Fig. 3a ). In contrast, caspase-3/7 were activated slightly earlier, which is in accordance with the relatively rapid clearance of full-length TDP-43 that carries the D89E mutation ( Supplementary Fig. 3a ). In addition, this result suggests that the generation of CTF35 is dispensable for the activation of caspases-3, -4 and -7. Similar to the D89E mutation, introduction of the D169G mutation either with or without the additional D89E mutation had no effect on the timing of caspase-4 activation ( Supplementary Fig. 3a,b ). In contrast, the activation of caspase-4 was inhibited almost completely by introduction of the D174A mutation, either with or without an additional D89E or D169G mutation, which is in accordance with the severe reduction of CTF25 production ( Supplementary Fig. 3a,b ). Furthermore, the subsequent activation of caspase-3/7 was weak and prolonged ( Supplementary Fig. 3c ). These results further support the idea that the initial cleavage of overexpressed TDP-43 after Asp174 is catalysed by activated caspase-4, which subsequently activates downstream caspase-3/7, which in turn accelerates the clearance of TDP-43 by fragmentation. Finally, we investigated whether specific inhibitors of the different caspases could block the generation of the CTFs. The inhibitor of caspase-3/7 significantly reduced the production of both CTF35 and CTF25 at 36 h, whereas the production of CTF25 at 0 h was unaffected ( Fig. 6b ). In contrast, the caspase-4 inhibitor significantly reduced both the production of CTF25 at 0 h and that of CTF35 and CTF25 at 36 h ( Fig. 6c ). Furthermore, inhibition of caspase-4 activity exacerbated the cell death induced by the overexpression of TDP-43 in both U2OS cells and hESC-derived motor neurons, which is similar to the effect obtained by blocking cleavage after Asp174 ( Fig. 6d,e ). Taken together, we concluded that caspase-4 is responsible for the initial cleavage of TDP-43 after Asp174, which is required for the avoidance of cell death induced by the overexpression of TDP-43. CTFs aggregate initially at the ER Given that caspase-4 is localized to the ER membrane [22] , we investigated whether TDP-43 and its derived fragments could be detected at the ER by staining the SNAP and Halo tags of SNAP-TDP-43(WT)-HTC at 0 h post induction and monitoring their localization for 72 h. At 12 h, SNAP-TDP-43(WT)-HTC was localized predominantly in the nucleus, whereas cytoplasmic inclusions that stained positively for the HaloTag, but negatively for SNAP, could be observed in the vicinity of the nucleus and within the ER at 36 h ( Fig. 7a and Supplementary Fig. 4a ). This timing is identical to that of the formation of insoluble CTFs ( Fig. 3a ). At 72 h, ~80% of SNAP-TDP-43(WT)-HTC had been cleared from the nucleus. However, the number and size of the HaloTag-positive cytoplasmic inclusions had increased, such that ~60% of the initial intensity of the intracellular HaloTag ligand was preserved ( Fig. 7a and Supplementary Figs 4b and 5 ). Some of these inclusions were both HaloTag- and SNAP-tag-positive and were detected outside the ER. These results suggest that aggregates of CTFs are formed initially at the ER; they then recruit full-length TDP-43 to form additional aggregates and spread to locations distant from the ER. Then, we examined whether caspase-4 was activated under ER stress as previously reported [22] . In addition to phosphorylated protein kinase-like ER kinase (PERK), an active form of PERK, the increased expression of ER markers, including Calnexin, IRE1α (inositol-requiring enzyme 1α) and PDI (protein disulfide isomerase) was observed after 72 h ( Fig. 7b ). These results suggest that caspase-4 is activated before the induction of ER stress, which might be stimulated by CTF aggregates that have accumulated in the ER. 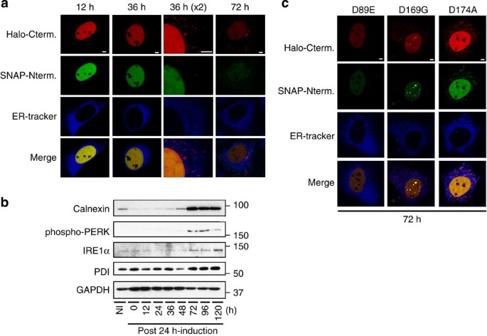Figure 7: CTF aggregates are formed initially at the ER. (a) Following induction of SNAP-TDP-43(WT)-HTC in U2OS cells for 24 h, the C terminus and N terminus were labelled with the ligands for HaloTag (top panel) and SNAP (second panel), respectively. ER was then stained with ER-Tracker (third panel). The distributions of SNAP-TDP-43(WT)-HTC and its fragments were monitored at the indicated time points. Merged fluorescent images are presented in the bottom panel. Sections of the images taken at 36 h have been enlarged ( × 2) and shown at increased intensity. Scale bars, 5 μm. (b) Transient expression of SNAP-TDP-43(WT)-HTC was induced with Dox for 24 h, and the expression of each ER stress marker indicated on the left was monitored at the indicated time points. GAPDH was used as the loading control. NI, no induction. (c) The distributions of SNAP-TDP-43-HTC with the point mutation D89E (left panel), D169G (middle panel), or D174A (right panel) and the corresponding fragments were monitored at 72 h after induction for 24 h in U2OS cells. Scale bars, 5 μm. Cterm, C-terminal; Nterm, N-terminal. Figure 7: CTF aggregates are formed initially at the ER. ( a ) Following induction of SNAP-TDP-43(WT)-HTC in U2OS cells for 24 h, the C terminus and N terminus were labelled with the ligands for HaloTag (top panel) and SNAP (second panel), respectively. ER was then stained with ER-Tracker (third panel). The distributions of SNAP-TDP-43(WT)-HTC and its fragments were monitored at the indicated time points. Merged fluorescent images are presented in the bottom panel. Sections of the images taken at 36 h have been enlarged ( × 2) and shown at increased intensity. Scale bars, 5 μm. ( b ) Transient expression of SNAP-TDP-43(WT)-HTC was induced with Dox for 24 h, and the expression of each ER stress marker indicated on the left was monitored at the indicated time points. GAPDH was used as the loading control. NI, no induction. ( c ) The distributions of SNAP-TDP-43-HTC with the point mutation D89E (left panel), D169G (middle panel), or D174A (right panel) and the corresponding fragments were monitored at 72 h after induction for 24 h in U2OS cells. Scale bars, 5 μm. Cterm, C-terminal; Nterm, N-terminal. Full size image Next we investigated how the cleavage-resistant mutations affected the localization of TDP-43 and its fragments. Introduction of the D89E mutation accelerated the shift of SNAP-TDP-43-HTC from the nucleus to cytoplasmic inclusions, which resulted in the absence of nuclear SNAP-TDP-43-HTC and the faint detection of cytoplasmic inclusions at 72 h ( Fig. 7c and Supplementary Figs 4c and 5 ). In contrast, introduction of the D169G mutation moderately decelerated the clearance of SNAP-TDP-43-HTC from the nucleus and led to the formation of large intranuclear inclusions that were positive for both the HaloTag and SNAP, although there was a simultaneous increase in the number of cytoplasmic inclusions at 72 h ( Fig. 7c and Supplementary Fig. 5 ). Introduction of the D174A mutation slowed the clearance of SNAP-TDP-43-HTC from the nucleus further, which is consistent with the previous finding that the majority of full-length SNAP-TDP-43-HTC with the D174A mutation remained at 96 h. Of note, the cytoplasmic inclusions were larger in number and size in the presence of the D174A mutant than in the presence of the wild-type protein or D169G mutant. In addition, in the former case, the inclusions spread reticularly within the ER, and a substantial proportion of the inclusions were both HaloTag- and SNAP-tag-positive ( Fig. 7c ). Taken together, these results suggest that although SNAP-TDP-43-HTC with the D174A mutation is transported to the ER, it is not recognized by caspase-4. Consequently, full-length SNAP-TDP-43-HTC accumulates within the ER and clearance of the protein from the nucleus is severely delayed. Necrosis is a predominant form of TDP-43-induced cell death Given that introduction of the D174A mutation induced severe and prolonged cell death, even though the activation of caspases was severely impaired ( Fig. 4a,b and Supplementary Fig. 3 ), we investigated the mechanism that underlies the cell death that is induced by the overexpression of TDP-43. Cells that stained positive with Ethidium Homodimer III (EthD-III), a marker of necrosis, were detected first at 24 h, whereas cells that were positive for Annexin V, a marker of apoptosis, or positive for both EthD-III and Annexin V could be observed at 48 h post induction of SNAP-TDP-43(WT)-HTC ( Fig. 8a ). This result suggested that the initial cell death is mediated through the necrotic pathway, but this is followed by apoptosis to some extent due to the activation of caspases. In contrast, in the presence of the D174A mutation, EthD-III-positive cells were detected more extensively than in the wild type, but Annexin V-positive cells were rarely observed at 48 h ( Fig. 8a ). This suggested that necrotic cell death was enhanced due to the delayed clearance of TDP-43 by the blockage of caspase-mediated TDP-43 fragmentation. There are two types of necrotic pathway, namely, necrosis and necroptosis, a programmed form of necrosis. We found that Necrostatin-1, a necroptosis-specific inhibitor, failed to restore cell viability, whereas NecroX-2, a necrosis-specific inhibitor, ameliorated the TDP-43-mediated cytotoxicity ( Fig. 8b,c ). This effect was especially evident in the D174A mutant, which further supports the theory that overexpression of TDP-43 induces necrosis. It was recently reported that the increased release of calcium ions from the ER is a driver of necrosis mediated by a mutant form of TDP-43 in C. elegans [23] . Consequently, we examined the effect of Dantrolene, which specifically inhibits the release of calcium ions from ER stores, on cell death induced by the overexpression of TDP-43. This analysis demonstrated that Dantrolene inhibited TDP-43-mediated necrosis significantly, especially when it was induced by the D174A mutation ( Fig. 8d ). These results suggested that the accumulation of TDP-43 in the ER might result in the release of calcium ions initially, which leads to necrosis. 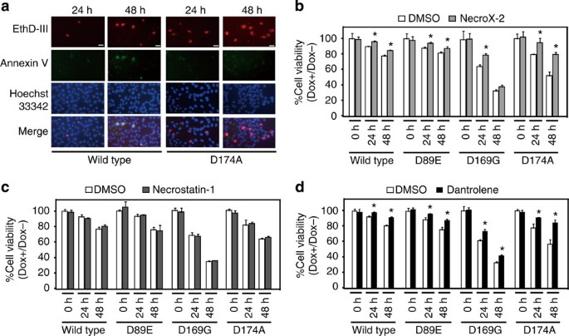Figure 8: Necrosis is the initial form of cell death that is induced by the overexpression of TDP-43. (a) Following the induction of SNAP-TDP-43(WT)-HTC or the D174A mutant in U2OS cells for 24 h, cells were stained with EthD- III (top panel), FITC-Annexin V (second panel) and Hoechst 33342 (third panel) at the indicated time points. Merged fluorescent images are presented in the bottom panel. Scale bars, 50 μm. Following the induction of SNAP-TDP-43(WT)-HTC or the mutants indicated at the bottom in U2OS cells for 24 h in the presence or absence of NecroX-2 (b), Necrostatin-1 (c) and Dantrolene (d), cell viability was quantitated at the indicated time points. The cell viability in the presence of Dox is plotted relative to that in the absence of Dox (mean±s.e.m.; *P<0.05,n=6 forbanddand 4 forc). The Mann–WhitneyU-test was used for all statistical analyses. DMSO, dimethylsulphoxide. Figure 8: Necrosis is the initial form of cell death that is induced by the overexpression of TDP-43. ( a ) Following the induction of SNAP-TDP-43(WT)-HTC or the D174A mutant in U2OS cells for 24 h, cells were stained with EthD- III (top panel), FITC-Annexin V (second panel) and Hoechst 33342 (third panel) at the indicated time points. Merged fluorescent images are presented in the bottom panel. Scale bars, 50 μm. Following the induction of SNAP-TDP-43(WT)-HTC or the mutants indicated at the bottom in U2OS cells for 24 h in the presence or absence of NecroX-2 ( b ), Necrostatin-1 ( c ) and Dantrolene ( d ), cell viability was quantitated at the indicated time points. The cell viability in the presence of Dox is plotted relative to that in the absence of Dox (mean±s.e.m. ; * P <0.05, n =6 for b and d and 4 for c ). The Mann–Whitney U -test was used for all statistical analyses. DMSO, dimethylsulphoxide. Full size image In contrast to the potent cytotoxicity that is induced by the overexpression of full-length TDP-43, it was reported that the overexpression of CTF35 or CTF25(D169) has very little or no ability, respectively, to induce cell death [15] . Furthermore, the expression of a CTF in the fly eye fails to induce neurodegeneration [12] . This evidence indicates that the regulation of the total amount of full-length TDP-43, rather than that of the CTFs, is a critical determinant of cell survival. Indeed, the expression of TDP-43 is elevated in neurons that have differentiated from patient-derived iPS cells that carry the M337V mutation [24] . Furthermore, TDP-43 proteins that are mutated have longer half-lives than the wild-type protein and these longer half-lives correlate with a more rapid onset of the disease [10] , [25] . In this study, we have demonstrated that the speed of clearance of full-length TDP-43 is a critical determinant of the severity of cytotoxicity and that the onset of cell death induced by the overexpression of TDP-43 occurs earlier than that of the formation of CTF aggregates, which might enhance cytotoxicity. Furthermore, it was thought that CTF25 is generated in parallel to CTF35 by caspase-3/7-mediated cleavage at minor sites. In addition, although the cytotoxic function of aggregated CTFs has been shown repeatedly [26] , [27] , the biological significance of the cleavage of TDP-43 has been poorly understood. However, the present study provides evidence that TDP-43 is cleaved after Asp174 by caspase-4, which results in the production of CTF25 before that of CTF35, and this event is required for the initiation of clearance of full-length TDP-43. Caspase-4 is bound to the ER membrane and is activated under ER stress [22] . Although the pharmacological induction of ER stress can cause TDP-43 to accumulate in the cytoplasm and promotes fragmentation, it has also been reported that overexpression of TDP-43 induces ER stress [15] , [28] , [29] , [30] . Furthermore, it has been shown that caspase-4 and markers of ER stress are upregulated in the spinal cords of patients with sporadic ALS [31] , [32] . However, the triggering factor and the order in which caspase-4 and ER stress are activated have remained unknown. We have identified caspase-4 as an initiator of TDP-43 clearance and found that its activation preceded the induction of ER stress. Furthermore, we found that CTF aggregates were formed initially at the ER, which suggests that the caspase-dependent cleavage of TDP-43 and the formation of aggregates occur sequentially at the ER. Therefore, we propose that caspase-4 plays a central role in monitoring the amount of TDP-43 in the ER by recognizing Asp174 and when the ER is overloaded with TDP-43, caspase-4 cleaves a small portion of TDP-43. This cleavage triggers the downstream caspase-3/7 pathway, which cleaves TDP-43 more efficiently and results in the formation of CTF aggregates and the induction of ER stress. Indeed, previous reports suggest that at least caspase-3 is activated by caspase-4 as a downstream effector caspase [33] , [34] . It is currently unknown why caspase-4 recognizes Asp174 more efficiently than Asp89 in vivo , even though caspase-4 can generate CTF35 more efficiently than CTF25 in vitro. Further study is required to elucidate this difference that might be attributed to differences in the accessibility of Asp89 and Asp174 to caspase-4 in the context of the ER, or alternatively other caspases such as caspase-3/7, which recognize Asp89 strongly, might competitively inhibit the access of caspase-4. The results of the present study demonstrate that the total molar amount of CTF35 and CTF25 is much less than that of the induced full-length TDP-43 at any time point during fragmentation. Although we cannot exclude the possibility that the majority of CTF35 and CTF25 is degraded quickly or that a large number of other CTFs are generated at low doses by cleavage at minor sites, it appears that caspase-dependent fragmentation is not the sole pathway for TDP-43 clearance. Indeed, the levels of CTFs are increased substantially in the presence of a proteasome inhibitor [10] . Furthermore, motor neuron-specific disruption of the ubiquitin–proteasome system (UPS) has been shown to induce locomotor dysfunction accompanied by progressive motor neuron loss and neuronal inclusions with TDP-43 in mice [35] . This evidence suggests that at least the UPS participates in the degradation of TDP-43. In addition, recent studies have reported that autophagy also contributes to the clearance of TDP-43, and although soluble TDP-43 is degraded primarily by the UPS, the clearance of aggregated TDP-43 requires autophagy [36] , [37] . Importantly, it has also been shown that caspase-3-dependent cleavage is required for the degradation of TDP-43 through the UPS and autophagy [37] . Overall, we propose that caspase-4-dependent cleavage is a required step for the initiation of TDP-43 clearance and activates downstream caspase-3/7, which induces the eventual degradation of TDP-43 by stimulating multiple pathways, such as the UPS and autophagy. Finally, the D169G mutation within TDP-43 is a unique ALS-linked mutation that resides outside the C-terminal GRD [4] . We have shown that introduction of the D169G mutation can moderately decrease the rate of clearance of full-length TDP-43, although Asp169 appears to be a very minor site for caspase-3/7-dependent cleavage. It has been reported recently that the D169G mutation does not affect nucleic acid binding to TDP-43 but does increase the thermal stability of the protein, which leads to resistance to thermal denaturation and an increased half-life [38] , [39] . This evidence suggests that the D169G mutation delays the clearance of full-length TDP-43 and induces severe cell death through two distinct mechanisms, that is, by blocking cleavage and increasing thermal stability. In addition, although our data show that CTF25(D169) is more prone to aggregation than CTF25(D174), the generation of CTF25(D169) is probably inhibited in patients with the D169G mutation. Therefore, although no cases of ALS carrying the D169G mutation have been reported on autopsy, the total amount of CTF25 aggregates in the affected regions of patients with this mutation might provide useful information regarding the role of CTF25 aggregates in the progression of neurodegeneration. In summary, we have identified Asp174 as a novel cleavage site in TDP-43. This cleavage is catalysed by caspase-4 at the ER, and generates CTF25 before the production of CTF35. In addition, we found that the caspase-4-mediated cleavage is required to initiate the clearance of full-length TDP-43, and inhibition of caspase-4 activity or introduction of a cleavage-resistant mutation at Asp174 results in the severe delay of TDP-43 clearance and prolonged necrotic cell death. Therefore, increasing caspase-4 activity or the rate of TDP-43 clearance might have therapeutic potential for ALS and FTLD. Antibodies and reagents The following primary antibodies were used: anti-HaloTag polyclonal antibody (pAb; 1:500, G928A, Promega), anti-SNAP-tag pAb (1:1,000, P9310S, NEB), anti-GAPDH mAb (1:50,000, M171-3, MBL), anti-TARDBP pAb (1:2,500, 10782-2-AP, ProteinTech), anti-TARDBP pAb for C terminus region (1:500, NB110-55376, NOVUS Biologicals), anti-TDP-43 N terminus (3-12) pAb (1:500, TIP-TD-P07, CosmoBio), anti-phospho TDP-43 (pS409/410-1) pAb (1:500, TIP-PTD-P01, CosmoBio), anti-cleaved caspase-4 (Gln81) pAb (1:250, GTX86890, GeneTex); anti-caspase-10 pAb (1:100, 3410-200, BioVision) anti-cleaved caspase-3 (Asp175) (5A1E) mAb (1:500, 9664), anti-cleaved caspase-6 (Asp162) pAb (1:500, 9761), anti-cleaved caspase-7 (Asp198) mAb (1:500, 8438), anti-cleaved caspase-8 (Asp391) mAb (1:500, 9496), anti-cleaved caspase-9 (Asp330) mAb (1:1,000, 7237) and anti-cleaved caspase-9 (Asp315) pAb (1:500, 9505), anti-Calnexin mAb (1:1,000, 2679), anti-IRE1α mAb (1:1,000, 3294), anti-phospho-PERK (Thr980) mAb (1:1,000, 3179), anti-PDI mAb (1:2,000, 3501; Cell Signaling Technology). Cell-permeable caspase-4 inhibitor (FMK005), caspase-3/7 inhibitor (3194-v), NecroX-2, Necrostatin-1 and Dantrolene were obtained from R&D Systems, PEPTIDE Institute Inc., Enzo Life Sciences, Millipore and Sigma, respectively, and dissolved in dimethylsulphoxide. HaloTag TMR Ligand and SNAP-Cell 505-Star were obtained from Promega and NEB, respectively. ER-Tracker Blue-White DPX, NucBlue Live ReadyProbes Reagent and ethidium homodimer-I (EthD-1) were obtained from Life Technologies. Cell culture Human U2OS cells were kindly provided by Professor Kazuhiro Iwai (Kyoto University). U2OS cells and ProAdhere 293T Cells (Applied Biological Materials) were maintained in Dulbecco’s modified Eagle’s medium supplemented with 10% Tet System Approved FBS (Clontech). Human ESC-derived Motor Neuron Progenitors were obtained from Lonza. The progenitor cells (8 × 10 4 cells per well) were cultured in NeuroBlast medium (Lonza) that contained 15 μg ml −1 Laminin (Roche) in 96-well plates coated with high molecular weight Poly- D -Lysine (Sigma) for 48 h to induce differentiation into motor neurons. Subsequently, half of the medium was replaced every other day with MotorBlast medium (Lonza). To analyse the effect of each reagent, the cells were cultured in the presence of each reagent (caspase-4 inhibitor (50 μM), caspase-3/7 inhibitor (50 μM), NecroX-2 (20 μM), Necrostatin-1 (50 μM) and Dantrolene (30 μM)), and the medium that contained the reagent was replaced every 24 h (refs 15 , 40 ). Plasmids and constructs To generate the expression construct for full-length TDP-43 tagged with SNAP at the N terminus and HaloTag at the C terminus (pSNAP-TDP-43(WT)-HTC), the coding region of TDP-43 was first amplified using the FALG-TDP-43 expression vector as the template [41] and inserted into the pFC14K vector (Promega) using the Sgf1 and EcoICR1 restriction sites to generate pFC14K-TDP-43-HTC. Next the TDP-43-HTC region was amplified and inserted into the pSNAP-tag(m) vector (NEB) using the Sbf1 and Not1 restriction sites. To generate the C terminus-truncated constructs (pSNAP-TDP-43(N1-89), pSNAP-TDP-43(N1-169) and pSNAP-TDP-43(N1-174)), the required regions were amplified using pSNAP-TDP-43(WT)-HTC as the template and inserted into pSNAP-tag(m) using the Sbf1 and Not1 restriction sites. Similarly, to generate the N terminus-truncated constructs (pFC14K-TDP-43(C90-414)-Halo, pFC14K-TDP-43(C170-414)-Halo, and pFC14K-TDP-43(C175-414)-Halo), the required regions were amplified using pSNAP-TDP-43(WT)-HTC as the template and inserted into pFC14K using the Sgf1 and EcoICR1 restriction sites. The N terminus- and C terminus-truncated constructs without tags were generated by amplifying the required regions using pSNAP-TDP-43(WT)-HTC as the template and inserting the fragments into pSNAP-tag(m) using the EcoRV and Not1 restriction sites. Digestion of pSNAP-tag(m) with EcoRV and Not1 removes the SNAP-tag so that the resulting construct is untagged. To generate pTRE-Tight-SNAP-TDP-43(WT)-HTC, the required regions were amplified using pSNAP-TDP-43(WT)-HTC as the template and inserted into the pTRE-Tight vector (Clontech) using the Kpn1 and Not1 restriction sites. To generate the mutant vectors, pTRE-Tight-SNAP-TDP-43(D89E)-HTC, pTRE-Tight-SNAP-TDP-43(D169G)-HTC, pTRE-Tight-SNAP-TDP-43(D174A)-HTC, pTRE-Tight-SNAP-TDP-43(D89E/D169G)-HTC, pTRE-Tight-SNAP-TDP-43(D89E/D174A)-HTC and pTRE-Tight-SNAP-TDP-43(D169G/D174A)-HTC, point mutations were introduced into pTRE-Tight-SNAP-TDP-43(WT)-HTC by site-directed mutagenesis using a QuikChange II Site-Directed Mutagenesis Kit (Agilent Technologies) with the appropriate primers. To generate the viral expression constructs, namely pLVSIN-CMV-SNAP-TDP-43(WT)-HTC and its mutants, the corresponding regions were inserted into the pLVSIN-CMV Pur vector (Clontech) using the XbaI and NotI restriction sites. To generate the wild-type and mutant pTNT-TDP-43-Myc constructs, the TDP-43 coding region was amplified with primers that contained the Myc sequence using pTRE-Tight-SNAP-TDP-43(WT)-HTC and its mutants as templates and inserted into the pTNT vector (Promega) using the Kpn1 and Not1 restriction sites. All point mutations were confirmed by sequencing each construct. Establishment of U2OS-derived stable cell lines Once they had reached ~90% confluence in 6-cm dishes, U2OS cells were transiently transfected with 4 μg each of pTRE-Tight-SNAP-TDP-43-HTC and the Tet-On Advanced vector (Clontech), and 400 ng of linear puromycin marker (Clontech) using Lipofectamine 2000 (Life Technologies). The day after transfection, the cells were transferred to fresh medium that contained 1.0 μg ml −1 puromycin (Sigma). After 3 weeks of puromycin-selective culture, puromycin-resistant single clones were isolated and expanded in 6-cm dishes. Protein expression was induced in the selected cells by supplementing the medium with 1.0 μg ml −1 Dox (Clontech). After 2 days of induction with Dox, the cells were collected and analysed for the expression of SNAP-TDP-43-HTC by western blotting. Western blot analysis Total cell lysates or affinity-purified proteins were separated by SDS–polyacrylamide gel electrophoresis, transferred to polyvinylidene difluoride membranes (Bio-Rad), and immunoblotted with antibodies using the SNAP i.d. 2.0 Protein Detection System (Millipore). The uncropped scans of the most important western blots are included in Supplementary Figs 6–19 . Purification of Halo-tagged proteins After the cells had been collected by centrifugation at 1,000 g for 5 min, the cell pellets were homogenized in cell lysis buffer (50 mM Tris-HCl, pH 7.4; 150 mM NaCl; 1 mM EDTA; 1% Triton-X-100) with protease inhibitor (Promega), and further digested by rotating at 4 °C for 30 min. After the whole-cell lysate (supernatant) had been collected by centrifugation at 15,000 g for 30 min at 4 °C, it was mixed with Halo-IP buffer (50 mM Tris-HCl, pH 7.4; 150 mM NaCl; 0.05% NP-40; 1 mM DTT) that had been equilibrated with HaloLink Resin (Promega) and rotated at 4 °C for 5 h to allow stable covalent binding of the Halo-tagged protein to the resin, in accordance with the manufacturer’s instructions. After the unbound protein had been removed by multiple washes, the bound proteins were dissociated from the resin by cleavage of the HaloTag from the target proteins with TEV protease. Analysis of the N-terminal cleavage sites The tag-free proteins were separated by SDS–polyacrylamide gel electrophoresis, transferred to a polyvinylidene difluoride membrane and stained with CBB R-250 (Bio-Rad). After the target bands had been excised, the N-terminal cleavage sites were determined by the Edman sequencing method using a Procise 494 HT Protein Sequencing System (Applied Biosystems) at APRO Science Inc. (Tokushima, Japan). Five to eight cycles of sequencing were performed for each sample. Sarkosyl-based fractionation of cells After the cells had been collected by centrifugation at 1,000 g for 5 min at 4 °C, the cell pellets were lysed in 3 × volumes of TS buffer (50 mM Tris-HCl, pH 7.4; 150 mM NaCl; 5 mM EDTA; 5 mM EGTA) with protease inhibitor, and separated by centrifugation at 150,000 g for 20 min at 4 °C as described previously [7] . The supernatant was defined as the TS-soluble fraction, and the pellets were solubilized in the same volume of 1% Triton-X-100 in TS buffer with protease inhibitor. Following centrifugation at 150,000 g for 20 min at 4 °C, the supernatant was collected as the TX-soluble fraction, and the pellets were further sonicated in TS buffer with 1% sarkosyl ( N -lauroylsarcosine, Sigma). After the TX-insoluble sonicates had been incubated at 37 °C for 30 min and centrifuged at 290,000 g for 20 min at 25 °C, the supernatant was collected as the Sarkosyl (Sark)-soluble fraction, and the pellets were dissolved in SDS sample buffer and boiled for 10 min. This SDS-soluble fraction was defined as the Sark-insoluble fraction [7] . In vitro caspase-cleavage assay The wild-type Myc-TDP-43 protein and its mutants were expressed using the TNT Quick Coupled Transcription/Translation system (Promega) in accordance with the manufacturer’s instructions. In brief, the transcription/translation reaction was performed at 30 °C for 90 min in a standard reaction mixture that contained reticulocyte lysate (20 μl), plasmid DNA (1 μg) and methionine (1 μl). The synthesized proteins (5 μl) were incubated at 37 °C for 4 h with 1 unit of recombinant human caspase-1–10 (BioVision) in a 10-μl reaction system that contained 50 mM HEPES, pH 7.2, 50 mM NaCl, 0.1% CHAPS, 10 mM EDTA, 5% glycerol and 10 mM DTT. Cell imaging Living U2OS cells grown on poly- D -lysine-coated glass bottom dishes were first labelled with SNAP-Cell Star 505 (NEB) at a concentration of 2 μM in complete medium for 30 min at 37 °C. After the medium had been replaced with complete medium that contained 1 μM HaloTag TMR ligand (Promega), the cells were incubated for 15 min at 37 °C. Cells that had been labelled with the ligands for SNAP and HaloTag were stained further with 1 μM ER-Tracker Blue (Molecular Probes) for 15 min at 37 °C. Images were taken with a × 100 objective lens on a FluoView FV1000 laser scanning confocal microscope (Olympus) using three detection channels (SNAP-Cell Star: 504 EX /532 EM ; HaloTag TMR ligand: 555 EX /585 EM ; ER-Tracker Blue: 374 EX /430 EM ). After labelling with HaloTag TMR ligand and ER-Tracker Blue, three-dimensional (3D) images were generated by reconstructing the piled images from 50 individual scans obtained at 0.5-μm intervals using Volocity 3D Imaging Analysis Software (PerkinElmer). The dead cells were detected using the Apoptotic/Necrotic/Healthy Cells Detection Kit (PromoKine) in accordance with the manufacturer’s instructions. In brief, the cells were incubated in staining solution that contained FITC-Annexin V (green), EthD- III (red) and Hoechst 33342 (blue) for 15 min at room temperature. After washing, images of the cells were captured using a fluorescence microscope (BZ-8000, KEYENCE). Although healthy cells were stained only with blue, necrotic cells were stained with both red and blue. Apoptotic cells were stained with both green and blue or with all three colours. Analysis of fluorescence intensity After incubation with 1 μM HaloTag TMR ligand for 15 min at 37°C, living cells were stained further with NucBlue Live ReadyProbes (Molecular Probes) for 20 min at 37°C. Images of the cells were taken with a × 20 objective using an IN Cell Analyzer 6000 confocal imaging system (GE Healthcare) through two detection channels (555 EX /585 EM and 374 EX /430 EM ). The fluorescence intensity of the HaloTag TMR ligand within the nucleus, which was defined as the area stained with NucBlue Live ReadyProbes, was analysed with the Developer Toolbox software (GE Healthcare). Lentiviral transduction pLVSIN-CMV-SNAP-TDP-43(WT)-HTC and its mutants were transfected into ProAdhere 293T Cells and the viral supernatants were collected using the Lenti-X HTX Packaging System (Clontech) in accordance with the manufacturer’s instructions. Then, the virus was concentrated 10-fold by precipitation with PEG 8000 (Sigma) overnight, dissolved in MotorBlast medium and kept at −80 °C until use. After the lentiviral titre had been measured using a Lenti-X qRT-PCR Titration Kit (Clontech), the medium that contained the virus (multiplicity of infection of 20) was mixed with Polybrene solution (at a final concentration of 8 μg ml −1 ) and then added to each individual well that contained hESC-derived motor neurons. Subsequently, the 96-well plates were centrifuged at 1,200 g for 100 min at 32 °C and the cells were incubated at 37 °C for 5–6 days. Cell viability assay Viability of U2OS cells was quantified by the WST-8 assay using a Cell Counting Kit-8 (Dojindo), which measures the ability of cells to convert water-soluble NADH into water-insoluble formazan. Cells were incubated with WST-8 reagent for 2 h at 37 °C, and the absorbance was measured at 450 nm by using a fluorometer (SH-9000Lab, CORONA ELECTRIC Co.). Cytotoxicity was measured by the lactate dehydrogenase (LDH) release assay using an LDH-Cytotoxic Test (Wako). Twenty-four hours before the assay, the cell medium was replaced with serum-free VP-SFM medium with GlutaMAX Supplement (Life Technologies). After the supernatant had been transferred to a new plate, the colour reagent was added and the samples were incubated for 30 min at room temperature. The reaction was terminated by the addition of the reaction terminator. The amount of LDH released from the dead cells was quantified by measuring the absorbance at 560 nm. The viability of hESC-derived motor neurons was quantified as described previously [42] with modifications. In brief, 5–6 days after transduction, the cells were first labelled with SNAP-Cell Star 505 for 30 min at 37 °C. After one wash with MotorBlast medium, the cells were further stained with 0.2 μmol l −1 EthD-1 for 30 min at 37 °C and subsequently washed twice with MotorBlast medium. The degree of cell viability was calculated by counting the number of SNAP-positive and EthD-1-negative neurons in each well (three wells in total) using a fluorescence microscope (BZ-8000, KEYENCE). Statistical analysis The Mann–Whitney U -test was used for all statistical analyses. All values are displayed as the mean±s.e.m. Statistical significance is displayed as P <0.05 (* and # ), P <0.01 (**) or P <0.001 (***). How to cite this article: Li, Q. et al. The cleavage pattern of TDP-43 determines its rate of clearance and cytotoxicity. Nat. Commun. 6:6183 doi: 10.1038/ncomms7183 (2015).